The amino-terminal structure of human fragile X mental retardation protein obtained using precipitant-immobilized imprinted polymers Flexibility is an intrinsic property of proteins and essential for their biological functions. However, because of structural flexibility, obtaining high-quality crystals of proteins with heterogeneous conformations remain challenging. Here, we show a novel approach to immobilize traditional precipitants onto molecularly imprinted polymers (MIPs) to facilitate protein crystallization, especially for flexible proteins. By applying this method, high-quality crystals of the flexible N-terminus of human fragile X mental retardation protein are obtained, whose absence causes the most common inherited mental retardation. A novel KH domain and an intermolecular disulfide bond are discovered, and several types of dimers are found in solution, thus providing insights into the function of this protein. Furthermore, the precipitant-immobilized MIPs (piMIPs) successfully facilitate flexible protein crystal formation for five model proteins with increased diffraction resolution. This highlights the potential of piMIPs for the crystallization of flexible proteins. Fragile X mental retardation protein (FMRP) is the main factor causing fragile X syndrome, which is the most common form of inherited mental retardation in humans with a frequency of 1:4,000 males and 1:6,000 females [1] , [2] , [3] . Recently, FMRP is found as a critical host factor used by influenza viruses to facilitate viral RNA replication [4] . Therefore, FMRP is an important drug target in protecting against influenza. Nonetheless, because of the highly flexibility, only two segments of FMRP’s structure (1−134 and 216−404 residues) have been characterized structurally [5] , [6] . The most powerful method for determining protein structure is X-ray crystallography, which relies on the availability of high-quality single crystals [7] . However, structural flexibility obfuscates the possibility to obtain high-quality crystals of flexible proteins using standard methods with many heterogeneous conformations adopted. Traditionally, proteins can be stabilized by adding precipitants into the protein solution [8] . This is because precipitants alter the protein–solvent or protein–protein contacts and give a supersaturated solution condition, and these agents help the protein molecules precipitate out of solution [9] . However, because of the presence of molecular thermodynamics and diffusion, free precipitant added to the solution cannot effectively unify the conformations of protein molecules containing flexible domains and linkers. Thus, flexible proteins crystallized out of solution in an attempt to form high-quality single crystals is a lengthy procedure and often with a low success rate. Here, we have developed an approach to introduce common protein precipitants, such as polyethylene glycol and ammonium sulfate, into molecularly imprinted polymers (MIPs), which we have named piMIP 1 and piMIP 2 , respectively, to facilitate flexible protein crystallization. MIPs that possess highly specific affinity for target molecules are formed in the presence of template molecules that are removed subsequently to leave complementary cavities. Thus, these prepared MIPs should improve effectively protein crystal yields that are challenging to obtain previously [10] , [11] , [12] , [13] , [14] . Currently, structure-unsolved flexible proteins are not successfully crystallized using MIPs, perhaps because conformational ordering of flexible proteins is not achieved. Here, we hypothesize that precipitant-immobilized molecular imprinted polymers (piMIPs) with active precipitant groups on the surface may combine the functions of MIPs and precipitants, that is, not only adsorb proteins from the solution leading to higher supersaturated conditions, but also interact with proteins assembled around them to form ordered crystals. The piMIPs are used to crystallize a flexible segment of FMRP, as well as five model proteins are also evaluated to test the role of the immobilized precipitant. Preparation and characterization of piMIPs After our extensive crystal screening of different segments, an unexploited segment of FMRP (1−209 residues) that crystallized was found and named FMRPΔ. However, following extensive optimization, X-ray diffraction of FMRPΔ was only to a resolution of 10 Å. Thus, to better understand the function and aid drug design, piMIPs were designed to facilitate FMRPΔ (abbreviated as F) crystallization ( Fig. 1 and Supplementary Fig. 1 ). To test the importance of immobilized precipitant on the MIPs, five model proteins, glucose isomerase (G), trypsin (T), proteinase K (P), lysozyme (L) and catalase (C), were also chosen and individual precipitants were used in accordance with their traditional crystallization trials, that is, (NH 4 ) 2 SO 4 for glucose isomerase and trypsin, Na/K tartrate for proteinase K, NaCl for lysozyme and polyethylene glycol (PEG) for catalase [15] , [16] , [17] , [18] , [19] . As shown in Supplementary Fig. 2 , poly(ethylene glycol)methyl ether acrylate containing a PEG group was used for the piMIP 1 series synthesis because of its !ideal water solubility and the accessibility of free radical polymerization. 2-Acrylamido-2-methyl-1-propanesulfonic ammonium (AMPSN) bearing a sulfonic ammonium group and a C=C bond was used for the piMIP 2 series. These two piMIP series were synthesized with the six proteins as templates, and named F-piMIP 1 , F-piMIP 2 , G-piMIP 1 , G-piMIP 2 , T-piMIP 1 , T-piMIP 2 , P-piMIP 1 , P-piMIP 2 , L-piMIP 1 , L-piMIP 2 , C-piMIP 1 and C-piMIP 2 . For the controls, MIPs without the precipitant component (that is, F-MIP 0 , G-MIP 0 , T-MIP 0 , P-MIP 0 , L-MIP 0 and C-MIP 0 ) were also prepared. Simultaneously, piNIPs were produced using the same procedure, but without proteins as the templates. Additionally, nonimprinted polymers (NIPs) without the precipitant component, namely NIP 0 , were also prepared as controls. To avoid any interference from the template in the crystallization trials, Fourier transform infrared (FT-IR) was used to monitor the complete removal of the template from piMIPs. As shown in Supplementary Fig. 3 , the spectrum of piMIP 1 was identical to the spectrum of piNIP 1 . Spectral comparison between piMIP 2 and piNIP 2 also demonstrated similar results. 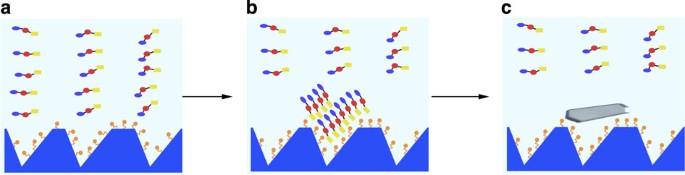Figure 1: Illustration of how the piMIPs play in protein crystallization. (a) Protein is flexible in solution. (b) piMIPs order the conformation of proteins with flexible loops at the surface. (c) Large single crystals grow out of the solution. To better compare the performance of different piMIPs and NIPs, the particle size distribution was examined, and results showed that the mean size of piMIPs and NIPs was 60−85 μm ( Supplementary Table 1 ). Figure 1: Illustration of how the piMIPs play in protein crystallization. ( a ) Protein is flexible in solution. ( b ) piMIPs order the conformation of proteins with flexible loops at the surface. ( c ) Large single crystals grow out of the solution. Full size image High-quality crystals of FMRPΔ obtained by piMIPs Bioinformatics analysis shows that the C-terminus of FMRPΔ is a highly flexible long loop [5] , [20] . piMIPs were used to obtain high-quality single crystals of FMRPΔ. Large single crystals were observed in the presence of F-piMIP 2 ( Supplementary Fig. 4a ) versus small crystals with F-piMIP 1 ( Supplementary Fig. 4b ). In addition, only small rod clusters ( Supplementary Fig. 4c–f ) were obtained with other piMIPs or CK, and no crystals with the MIP 0 or NIPs. As shown in Fig. 2 , the resolution of FMRPΔ crystals formed in the presence of F-piMIP 2 was 3.0 Å, whereas the best resolution of 10 Å was obtained for crystals without MIPs ( Table 1 ). 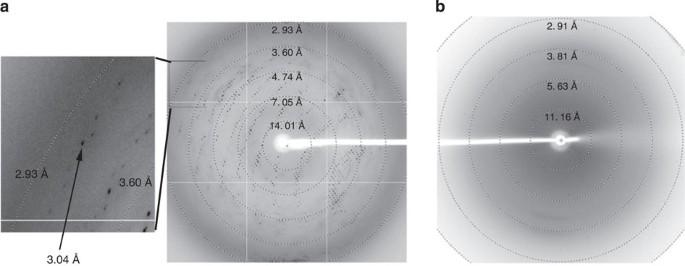Figure 2: X-ray diffraction images from FMRPΔ. (a) In the presence of F-piMIP2and (b) without any polymers. High-resolution regions inaare enlarged and brightened. Figure 2: X-ray diffraction images from FMRPΔ. ( a ) In the presence of F-piMIP 2 and ( b ) without any polymers. High-resolution regions in a are enlarged and brightened. Full size image Table 1 Crystallization results of molecularly imprinted polymers with cognate or noncognate proteins at metastable conditions. Full size table Structure of human FMRPΔ The molecular replacement method was used successfully with the structure of FXR1 (Protein Data Bank (PDB) accession number 3O8V ) [21] as the model to solve the human FMRPΔ structure after this approach failed using the previously reported FMRP NMR structure (residues: 1−134, PDB: 2BKD) [5] and other Tudor proteins as the search model. The final structure of the human FMRPΔ determined in this study contains four protein molecules (residues 1−200; Fig. 3a , Supplementary Fig. 5 and Supplementary Movie 1 ), 2 Tris ions and 171 water molecules in the asymmetric unit. The C-terminal nine residues were omitted from the structure because of the lack of electron density. The solvent content is as high as 78%. The four FMRPΔ structures are identical, with a root-mean-square deviation (RMSD) of 0.9 Å between their C-alpha atoms ( Table 2 ). Each FMRPΔ molecule contains three domains named Tudor1 (also termed NDF1 (ref. 5 ), residues 1−48; Fig. 3b , yellow), Tudor2 (also termed NDF2 (ref. 5 ), residues 61−108; Fig. 3b , blue) and a novel KH0 domain ( Fig. 3b , cyan). Overall, the three domains are stabilized with inter-domain polar and hydrophobic interactions, and form an integral structure. Moreover, there are two long inter-domain flexible loops and ten small labile loops. Interestingly, an intermolecular disulfide bond between the Cys99 residues in the Tudor2 domain of two FMRP monomers is found ( Fig. 3a and Supplementary Movie 1 ). 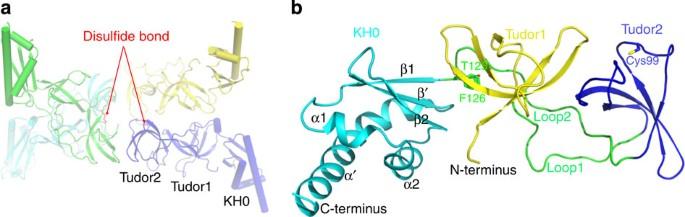Figure 3: Overall structure of human FMRPΔ. (a) Ribbon representation of the human FMRPΔ tetramer structure in the asymmetric unit. The four subunits are coloured green, cyan, yellow and blue, respectively. The two intermolecular disulfide bonds between Cys99 are highlighted in red. (b) Domain organization of human FMRPΔ depicting the Tudor1 (yellow), Tudor2 (blue), the new-found KH0 (cyan) and two long flexible loops between them. The residue Cys99, N-terminus, C-terminus and the loops are labelled. Figure 3: Overall structure of human FMRPΔ. ( a ) Ribbon representation of the human FMRPΔ tetramer structure in the asymmetric unit. The four subunits are coloured green, cyan, yellow and blue, respectively. The two intermolecular disulfide bonds between Cys99 are highlighted in red. ( b ) Domain organization of human FMRPΔ depicting the Tudor1 (yellow), Tudor2 (blue), the new-found KH0 (cyan) and two long flexible loops between them. The residue Cys99, N-terminus, C-terminus and the loops are labelled. Full size image Table 2 Data collection and refinement statistics of human FMRPΔ*. Full size table piMIPs do not alter Tudor1 and Tudor2 structures The N-terminal part of FMRPΔ contained two Tudor domains, Tudor1 and Tudor2. Both Tudor1 and Tudor2 fold into barrel-like four-stranded antiparallel β-sheets and pack against each other via an inter-domain 12-residue linker termed loop1 ( Fig. 3b , green). Loop2 (residues 108−126, Fig. 3b , green), which joins the Tudor2 to the C-terminal part of FMRPΔ, has strong interactions with Tudor1. The fold of Tudor1 and Tudor2 in this study adopts the same fold as reported in the NMR structure [5] with a low RMSD of 1.5 and 1.8 Å, respectively ( Fig. 4a left and middle panel). Moreover, the overall structure of Tudor1 and Tudor2 in this study is most similar to the structure of FXR1 (PDB: 3O8V (ref. 21 ), Z score, 15.7; RMSD, 1.2 Å; Supplementary Fig. 6 ) as searched by the Dali server [22] . Therefore, the piMIPs used in this study did not affect the protein structure. Intriguingly, the overall structure of the two Tudor domains determined in this study differs greatly from that of the NMR structure [5] with a high RMSD of 3.2 Å ( Fig. 4a right panel). This is because the NMR structure [5] and the present crystal structure differ greatly in the conformations of the loops and the relative orientation of these two Tudor domains. The large difference suggests that the structure of the FMRPΔ is highly flexible, further supporting our hypothesis that piMIPs can greatly stabilize flexible conformations. Meanwhile, the crystal structure determined in this study may be more close to the full-length FMRP structure, because it has an extensive C-terminal part that stabilizes the two Tudor domains. 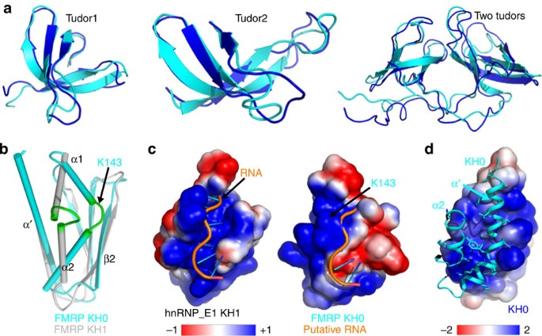Figure 4: Structure analysis of three domains of FMRPΔ. (a) Superposition of Tudor1 domain, Tudor2 domain and the structure comparison among the two Tudor domains in this study (light blue) and the solved NMR structure5(dark blue). (b) Superposition of the KH0 and KH1 domain of human FMRP. KH0 is coloured cyan and KH1 is coloured grey. For convenience, only β2, α1, α2 and α′ of KH0 are labelled. The highly conserved GXXG motif in KH1 (here is GTHG) and the corresponding part (K143) in KH0 are both coloured in green. (c) Electrostatic surface representation of hnRNP_E1-RNA complex (PDB accession number3VKE) and superimposition of FMRPΔ KH0 domain with hnRNP_E1-RNA complex. hnRNP_E1 is hidden but RNA is shown in stick. α1, K143 and α2 in the KH0 domain of human FMRPΔ will block the binding of single-strand nucleic acid and the nucleic acid will crash the KH0 domain. (d) Interaction between KH0 domain and symmetric KH0 domain in the large positive surface. Figure 4: Structure analysis of three domains of FMRPΔ. ( a ) Superposition of Tudor1 domain, Tudor2 domain and the structure comparison among the two Tudor domains in this study (light blue) and the solved NMR structure [5] (dark blue). ( b ) Superposition of the KH0 and KH1 domain of human FMRP. KH0 is coloured cyan and KH1 is coloured grey. For convenience, only β2, α1, α2 and α′ of KH0 are labelled. The highly conserved GXXG motif in KH1 (here is GTHG) and the corresponding part (K143) in KH0 are both coloured in green. ( c ) Electrostatic surface representation of hnRNP_E1-RNA complex (PDB accession number 3VKE ) and superimposition of FMRPΔ KH0 domain with hnRNP_E1-RNA complex. hnRNP_E1 is hidden but RNA is shown in stick. α1, K143 and α2 in the KH0 domain of human FMRPΔ will block the binding of single-strand nucleic acid and the nucleic acid will crash the KH0 domain. ( d ) Interaction between KH0 domain and symmetric KH0 domain in the large positive surface. Full size image KH0 is a novel subtype of K-Homology domain Interestingly, an uncharacterized domain ( Fig. 3b , cyan, residues 127−200) was found in the FMRPΔ C-terminal part ( Supplementary Movie 1 ). We next analysed the existence of structural similarity between this domain and other proteins by scanning the PDB using the DALI server [22] . The structure of the FMRPΔ C-terminal domain was found to be most similar ( Z score, 4.7; RMSD, 3.1 Å) to the first K-homology (KH) domain of human heterogeneous nuclear ribonucleoprotein E1 (hnRNP_E1) [23] , the first KH domain of human Vigilin (PDB: 2CTK, Z score, 4.5; RMSD, 3.5 Å) and the third KH domain of human RNA-binding protein Nova-2 ( Z score, 4.3; RMSD, 3.8 Å) [24] . These protein domains belong to the type I KH domain family, which has a C-terminal β-α extension [25] . The DALI search also revealed that this new-identified domain adopts the same fold as the other two known KH domains (KH1 and KH2) of FMRP [6] . Moreover, this new-found KH domain has a Z score of 4.1 and a RMSD of 2.9 Å with the other two KH domains of FMRP [6] . Therefore, we named this novel KH domain KH0, because the domain is at the N terminus of KH1. KH0 consists of a β-sheet composed of three antiparallel strands (β1, β2 and β′), which is abutted by three α-helices (α1, α2 and α′; Fig. 3b ) with the topology β1-α1-α2-β2-β′-α′ found in type I KH domains [25] . Our structural analysis is consistent with the observation that KH domains of eukaryotic proteins are exclusively type I [25] , [26] . Strikingly, sequence alignment of KH0 with other KH domains [6] , [24] showed relatively low similarity ( Supplementary Fig. 7 ). In contrast to other known KH domains, the FMRPΔ KH0 domain has several significant differences. First, the GXXG motif in the loop between α1 and α2 is highly conserved in other KH domains, but it is replaced by a single residue K143 in the KH0 domain. Second, two hydrophobic residues underlined in the IGXXGXXI motif are conserved among most KH domains [25] (red asterisk in Supplementary Fig. 7 ), whereas the KH0 domain does not have the corresponding hydrophobic residues. Accordingly, our structure confirms that these features make a major difference. On the one hand, the position of α1-loop-α2 in the KH0 domain is significantly different to the same loop in other KH domains [25] , such as the KH1 domain of FMRP or hnRNP_E1 ( Fig. 4b,c ). Moreover, the structures of hnRNP_E1 with and without RNA show no observed changes in the conformation of α1-loop-α2 upon ligand binding [23] . Therefore, the position of the α1-loop-α2 in the FMRP KH0 domain would repel the putative single strand nucleic acid if it shares the same binding mode as hnRNP_E1 ( Fig. 4c right panel). Conversely, in the corresponding RNA-binding position of the hnRNP_E1 KH1 domain ( Fig. 4c left panel), no continuous positive charge concave is found in the FMRP KH0 domain ( Fig. 4c right panel). In summary, these differences strongly suggest that the functions of the FMRP KH0 domain and its mode of interaction with putative binding partners may be quite different from other KH domains. Hence, KH0 may be classified as a novel subtype of the KH domains. FMRPΔ mainly exists as dimers in solution As shown in Fig. 3a , the solved FMRPΔ structure contains four protein molecules. This raised the question to whether FMRPΔ exists as a tetramer in solution. To ascertain the oligomeric state of FMRPΔ in solution, we employed two methods: gel filtration and analytical ultracentrifugation. We first evaluated the oligomeric state of FMRPΔ by gel filtration on a calibrated Superdex 75 10/300 column. The averaged molecular mass of the elution peak was 58.6 kDa ( Fig. 5a ), slightly larger than the value expected for the dimer (48 kDa). This observation is consistent with the apparent molecular weight of FMRPΔ shown by SDS–polyacrylamide gel electrophoresis ( Supplementary Fig. 8 ) being ~29 kDa, also larger than the calculated molecular weight (24 kDa). Moreover, analytical ultracentrifugation was used to assess the states of wild-type FMRPΔ in solution. The sedimentation velocity (SV) results indicated that FMRPΔ exists mainly as a dimer, but contains ~10% monomer and almost no tetramer ( Fig. 5b ). 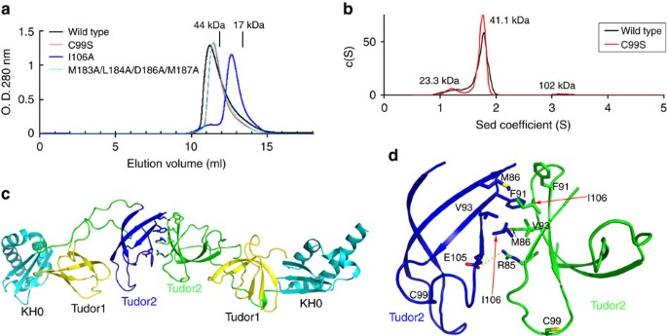Figure 5: Ile106 is a key residue for FMRPΔ dimerization. (a) Elution profiles of FMRPΔ mutants in a Superdex 75 10/300 GL column. Wild type, C99S, I106A and M183A/L184A/D186A/M187A quadruple mutants are coloured black, red, blue and cyan, respectively. Peak positions for two standard proteins are marked by lines on the top. (b) Analytical ultracentrifugation of FMRPΔ wild type and C99S Mutant. c(s) distribution from sedimentation velocity analytical ultracentrifugation experiments performed at 0.2 mM protein concentration. FMRPΔ almost exists as a dimer in solution. The peak of FMRPΔ C99S mutant is sharper. (c) The dimer based on Tudor2 domains and (d) the interactions between two Tudor2 domains. Two Ile106 are in the centre of the hydrophobic interface. Figure 5: Ile106 is a key residue for FMRPΔ dimerization. ( a ) Elution profiles of FMRPΔ mutants in a Superdex 75 10/300 GL column. Wild type, C99S, I106A and M183A/L184A/D186A/M187A quadruple mutants are coloured black, red, blue and cyan, respectively. Peak positions for two standard proteins are marked by lines on the top. ( b ) Analytical ultracentrifugation of FMRPΔ wild type and C99S Mutant. c(s) distribution from sedimentation velocity analytical ultracentrifugation experiments performed at 0.2 mM protein concentration. FMRPΔ almost exists as a dimer in solution. The peak of FMRPΔ C99S mutant is sharper. ( c ) The dimer based on Tudor2 domains and ( d ) the interactions between two Tudor2 domains. Two Ile106 are in the centre of the hydrophobic interface. Full size image Careful structure analysis showed that there are three types of dimer in the solved FMRPΔ structure ( Fig. 3a and Supplementary Fig. 9 ). The first dimer is the disulfide bond-based dimer ( Fig. 6a ) with an interface area of 508.4 Å 2 , as determined by PISA [27] . The second one is the Tudor2 domain-based dimer, formed by two adjacent Tudor2 domains ( Figs 5c and 6b ). The interface area is 506.8 Å 2 . The third one is the KH0 domain-based dimer ( Figs 4d and 6c and Supplementary Fig. 9 ), formed by the KH0 domain and the symmetric KH0 domain with an interface area of 897.3 Å 2 , which is 80% larger than the above two dimeric interfaces. There are extensive hydrophobic and hydrogen bond interactions among the four helices (two α′ and two α2) between two KH0 domains ( Supplementary Fig. 9a,b ). 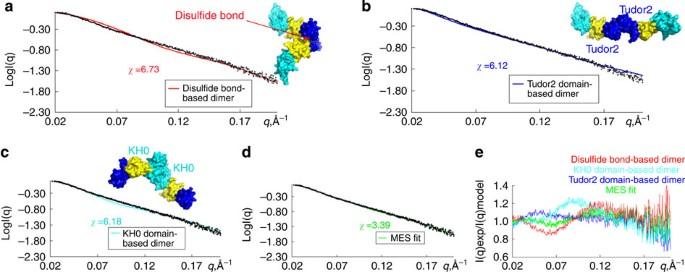Figure 6: FMRPΔ has several kinds of dimers in solution. Comparison of experimental data and calculated scattering profiles for wild-type FMRPΔ. Experimental data are represented in black dots. (a) The theoretical scattering curves of disulfide bond-based dimer (red), (b) Tudor2 domain-based dimer (blue), (c) KH0 domain-based dimer (cyan) and (d) the assembly from MES fit (green) are shown. (e) Residuals of four models calculated asI(q)experimental/I(q)model. Figure 6: FMRPΔ has several kinds of dimers in solution. Comparison of experimental data and calculated scattering profiles for wild-type FMRPΔ. Experimental data are represented in black dots. ( a ) The theoretical scattering curves of disulfide bond-based dimer (red), ( b ) Tudor2 domain-based dimer (blue), ( c ) KH0 domain-based dimer (cyan) and ( d ) the assembly from MES fit (green) are shown. ( e ) Residuals of four models calculated as I ( q ) experimental / I ( q ) model . Full size image To know which dimer FMRPΔ adopts in solution, we mutated several key residues in the above two larger interfaces. The disulfide bond C99S mutant resembles the FMRPΔ wild-type, as evaluated by gel filtration and analytical ultracentrifugation ( Fig. 5a,b ). Moreover, the addition of a high concentration of reducing reagents, such as dithiothreitol and tris(2-carboxyethyl)phosphine (TCEP), to the wild-type protein does not obviously change the oligomeric state in the sieve column. According to the interface between the two KH0 domains ( Supplementary Fig. 9b ), residues Met183, Leu184, Asp186 and Met187 are important for hydrophobic and hydrophilic interactions. However, the M183A/L184A/D186A/M187A quadruple mutant (KH0 mutant) was found to also not change its oligomeric state in the sieve column ( Fig. 5a ). Interestingly, the peak widths at half-peak height are significantly reduced, the peaks become sharper for both C99S and KH0 mutants. We further mutated the residues at the interface formed by two adjacent Tudor2 domains ( Figs 5c and 6b ). The interface is mainly formed by hydrophobic residues Phe91, Met86, Val93 and Ile106 from two Tudor2 domains. In addition to the hydrophobic interactions, there is an electrostatic interaction between Arg85 and Glu105. Structural analysis shows that the two Ile106 residues are in the centre of the hydrophobic interaction. Therefore, mutation of Ile106 to a small residue should greatly reduce the dimeric interaction. To validate this hypothesis, we mutated Ile106 to alanine. As expected from the structural observations, the molecular weight corresponding to the elution peak of the FMRPΔ I106A mutant was one-half of the wild type. This indicates that most of the I106A mutant is monomeric in solution ( Fig. 5a blue line). Therefore, Ile106 is a key residue for FMRPΔ dimerization. This observation confirms that the Tudor domain is a platform for protein–protein interactions [5] . FMRPΔ dimer has several kinds of conformations in solution The above I106A mutagenesis results show that the Tudor2 domain-based dimer is the major dimer conformer in solution. This raises the question to whether both the disulfide bond and the interface between two KH0 domains are crystallization artefacts. The wild-type FMRPΔ dimer was further purified by the sieve column to remove the monomer species. Small-angle X-ray scattering analysis (SAXS) was conducted to analyse the component of dimers in solution. SAXS is a powerful tool for structure validation and the quantitative analysis of flexible systems, and is highly complementary to the high-resolution methods of X-ray crystallography and NMR. Among the three fit SAXS profiles, the Tudor2 domain-based dimer ( Fig. 6b ) is the best-fit dimer. However, the theoretically calculated SAXS profile from any dimer model does not agree well with experimental data ( χ =6.12, 6.18 and 6.73; Fig. 6a–c ) and the errors are large ( Fig. 6e ). Thus, minimal ensemble search (MES) was applied to select a subset containing one to three dimers to best fit the experimental data [28] . The method is very useful in the analysis of conformers in solution. An ensemble containing all three conformers fits the data significantly much better ( χ =3.39; Fig. 6d ) than the single best-fit dimer ( χ =6.12). The observation is consistent with the experimental result that the dimer still exists in the I106A mutant ( Fig. 5a blue line). The results suggest that FMRPΔ has several kinds of dimeric conformers in solution, in which the major dimer species involves the Tudor2 domains as the interaction interface. We further analysed the dimer component of the C99S mutant by SAXS. The single best-fit model ( χ =3.46) is also the Tudor2 domain-based dimer ( Supplementary Fig. 10a ). The MES approach using three dimer models did not improve the fit ( χ =3.44) obviously ( Supplementary Figs 9d and 10c ). In the optimized mixture, the proportion of the Tudor2 domain-based dimer and the KH0 domain-based dimer ( Supplementary Fig. 10b ) are 94% and 6%, respectively, whereas no disulfide bond-based dimer is found. For the same single best-fit model, the fit of the experimental data and calculated scattering profiles of the wild-type FMRPΔ ( χ =6.12) is obviously worse than that of the C99S mutant ( χ =3.46; comparing Fig. 6b with Supplementary Fig. 10a ), implying that the disulfide bond exists in the wild-type protein. Thus, several FMRPΔ dimer species present in the solution, which is consistent with the size exclusion result of the FMRPΔ mutants. Thus, FMRPΔ has several kinds of dimeric conformations in solution. The calculated interface area of the Tudor2 domain-based dimer is 506.8 Å 2 , much lower than the value of 1,600±400 Å 2 that is generally believed to be of physiological significance [29] . Thus, the small interface between the two Tudor2 domains appears to be insufficient to maintain all dimers in this type. Moreover, this conclusion is consistent with the above mutagenesis data that the peaks are sharper and the peak widths at half peak height are greatly reduced after the C99S or KH0 mutation, and the dimer still exists in the I106A mutant ( Fig. 5a, b ). Therefore, our data confirmed that the disulfide bond formed by two Cys99 residues and the KH0 domain plays some roles in FMRP oligomerization. The performance of piMIPs in the five model proteins Table 1 showed that protein crystals were observed in their cognate piMIPs ( Supplementary Fig. 11 ) and in some noncognate piMIPs, MIP 0 and piNIPs but were not observed in the NIP 0 and CK (without any polymers) samples under metastable conditions ( Table 1 ). For glucose isomerase, a protein that readily crystallizes, crystals were found to form using any kind of piMIPs or MIP 0 . However, in the absence of the immobilized precipitant, the diffraction resolution of the crystals formed with MIP 0 (3.0 Å) was much lower than the resolution obtained with piMIPs (2.0 Å; Table 1 ). We also found that glucose isomerase crystals formed in the presence of piNIP 2 , but not in the CK and NIP 0 conditions. Moreover, because of the lower affinity of non-cognate piMIPs, crystals formed at a higher supersaturation condition than that observed with cognate piMIPs, thereby producing poorer and smaller crystals. This was also certified by comparing the diffraction resolution limit of crystals formed in the presence of G-piMIPs (2.0 Å) and other piMIPs (only 3.0 Å). Proteinase K also yielded crystals in the presence of P-piMIPs as well as other piMIPs and MIP 0 . However, the diffraction resolution limit was 1.06 Å ( Supplementary Fig. 12a ), 1.2 Å ( Supplementary Fig. 12b ) and 1.4 Å, respectively. Trypsin crystals appeared within 2 days in the presence of T-piMIP 2 (1.2 Å, Supplementary Fig. 12c ) and within 3−7 days with piNIP 2 (1.37 Å) and T-MIP 0 (1.42 Å). Lysozyme formed crystals within 24 h in the presence of L-piMIP with a diffraction resolution limit of 1.4 Å ( Supplementary Fig. 12d ), which was better than that observed with G-piMIP or MIP 0 (1.6 Å). Catalase yielded single large crystals within 3 days in the presence of C-piMIP 1 with a diffraction resolution at 2 Å versus smaller crystals in the presence of G-piMIP 1 (3.17 Å) and piNIP 1 (3.6 Å). No catalase crystals were observed with MIP 0 . In addition, from Table 1 we found that trypsin crystals appeared only in the presence of T-piMIP 2 and not in the presence of T-piMIP 1 . For catalase, crystals were only yielded with C-piMIP 1 and piNIP 1 but not with C-piMIP 2 and piNIP 2 . Nevertheless, for lysozyme and proteinase K, although both cognate piMIP 1 and piMIP 2 induced crystal growth, piMIP 2 produced crystals faster than piMIP 1 where the immobilized precipitant was mismatched with the free precipitant. In the present study, we successfully used the piMIPs method to obtain high-quality single crystals of a structure-unsolved flexible N-terminus of FMRPΔ, demonstrating the superior performance of cognate piMIPs in crystal growth for highly flexible proteins. Structure comparison of Tudor1 and Tudor2 domains reveals that the piMIPs method does not alter protein structures. FMRPΔ mainly exists as dimers in solution with several dimer species present ( Fig. 6 ). The present study paves the way to further study the self-association property of this key protein. Interestingly, an intermolecular disulfide bond between the Tudor2 domains of two FMRPΔ monomers was found in the crystal structure ( Fig. 3a ), and the existence of the disulfide bond in solution and the effect of C99S mutation on FMRP were confirmed by SAXS, gel filtration and analytical ultracentrifugation ( Fig. 5a,b ). The FMRP protein is mainly expressed in the cytoplasm and plays a role in the transport of mRNA from the nucleus to the cytoplasm [30] , [31] . In general, cytoplasmic proteins do not contain disulfide bonds. However, protein disulfide bond formation in the cytoplasm was observed during oxidative stress [32] . Interestingly, FMRP is identified as a chromatin-binding protein that functions in the DNA damage response [33] and oxidative DNA damage is an inevitable consequence of cellular metabolism [34] . Thus, dynamic regulation of FMRP disulfide bond formation may be involved in the oxidative DNA damage response. Moreover, disulfide bonds play important roles in the regulation of protein function and cellular stress responses, such as karyopherin-dependent nuclear transport [35] . Thus, our finding provides initial evidence that disulfide bonds may play a role in FMRP oligomerization and function. We also find that the C-terminal newly solved KH0 domain is a novel subtype KH domain. Sequence alignment of KH0 with other KH domains [6] , [23] , [24] shows relatively low similarity ( Supplementary Fig. 7 ). Structural analysis suggests that the KH0 domain may have a different function to that of regular KH domains ( Fig. 4b ). First, it does not resemble other KH domains’ interaction with single-stranded RNA (ssRNA) via the consensus GXXG motif [1] , [23] , because α1, K143 and α2 in the KH0 domain of human FMRPΔ will block the binding of ssRNA due to the steric hindrance and the repulsive electrostatic interactions. This expands our understanding of the selective RNA-binding function [1] , [23] , [36] of FMRP, because this is the first report of a novel KH domain ( Fig. 4c ). Second, a large positive charge surface on the KH0 domain was found ( Fig. 4d ). Third, the interaction between two adjacent KH0 domains was confirmed by SAXS and gel filtration. The interface area between two KH0 domains is 80% larger than the other two interfaces observed in two adjacent FMRPΔ molecules. Thus, the large size of the interface surface, the large positive charge surface and the observation of the KH0 domain-based dimer strongly suggests that the KH0 domain may provide a platform for protein–protein or protein–nucleic acid interactions. Even more dramatic is that the KH0 domain is involved in multiple protein–protein interactions. For example, it has been reported that residues 173−218 of FMRP are responsible for the interaction of FMRP with Cytoplasmic FMRP Interacting Protein 1 and 2 (refs 37 , 38 ). Interestingly, this part contains the α′ helix of the KH0 domain. Moreover, residues 171−211 are sufficient for FMRP interaction with FXR2, suggesting that the KH0 domain plays an important role in binding FXR family members [39] . Residues 66−134 of FMRP, which covers the N-terminus of KH0 (residues 127−134), has been also defined as an interacting site with the 82-kDa FMRP Interacting Protein and Nuclear FMRP Interacting Protein 1 (ref. 40 ). In addition, because of the large positively charged surface, the KH0 domain may be able to bind double-stranded RNA. For example, it was reported that this KH0 domain is essential for binding brain cytoplasmic RNA 1 (refs 41 , 42 ). Our results reveal that a newly identified domain, KH0, accounts for the ability of FMRP to interact with proteins or nucleic acids with a fresh perspective. It is well known that KH domains bind ssRNA via the consensus GXXG motif and functions in ssRNA recognition [25] . Taken together, this discovery of the KH0 domain indicates a new function of the KH domain, which requires further investigation. Recently, two papers [33] , [43] showed that the FMRP developmentally delayed patient mutation R138Q affects its nucleosomal binding and thus loses its function in DNA damage response processes. Analysis of the KH0 domain structure reveals that residue R138 forms an electrostatic interaction network with three negative residues in the loops between β1 and α1, and β2 and β′ ( Supplementary Fig. 13 ). Mutation of R138 with glutamine, will likely disrupt this electrostatic interaction network and the surface-positive charge, and thus may affect protein–protein interactions with its partners. Thus, FMRP may provide several flexible platforms for protein–protein or protein–nucleic acid interactions, enabling self-association and interactions with other proteins or nucleic acids, such as the nucleosome, FXR2, ribosome and brain cytoplasmic RNA 1. Our structure may help our understanding of the mechanism of intracellular localization of FMRP, because it reveals that residues 127−200 of FMRP constitute an independent KH0 domain with a compact fold. A nuclear localization function between residues 117 and 184 had been mapped using chicken muscle pyruvate kinase as a reporter protein [30] , and it was concluded that the activity of the nuclear localization sequence (NLS) is localized between residues 115−150 and the region between residues 151−196 could reinforce NLS activity [31] . However, FMRP lacks a NLS [5] , [30] , [31] . These experimental results, together with the above discussion, suggest that the KH0 domain may provide a platform for interaction of FMRP with nuclear components. The nuclear localization function of FMRP may be achieved by interacting with particular proteins containing a nuclear localization signal. In this regard, residues T125 and P126 ( Fig. 3b ) of FMRP may play important roles. It has been reported that the T125A/F126A double mutant destabilizes the Tudor fold and causes a different cellular localization of FMRP [5] . Structure analysis shows that residues T125 and P126 form strong hydrophobic interactions with the KH0 and Tudor1 domains. Here, it is proposed that residues T125 and P126 hold the KH0 domain and the two Tudor domains together to interact with particular nuclear components or proteins containing a NLS and then function to control the intracellular location of FMRP. Furthermore, because KH0 and the known KH1-KH2 domains of FMRP are adjacent in sequence and there is a nine-residue flexible loop between them, all three domains build a tandem KH domain architecture. Thus, we postulate that the relative orientation of the KH0 and KH1-KH2 domains in full-length FMRP may resemble some analogous tandem KH domain-containing proteins like bacterial protein NusA [44] , [45] , and play a similar role in the cell. In a parallel study, the crystal structure of FMRP (1–213) was also reported [46] . Yet, the structure was obtained using protease digestion and the maximum resolution of wild-type FMRP was 3.19 Å. The amino-terminal terminus of FMRP contains an integral tandem Agenet (Tudor) and a novel KH motif. The overall structure of monomeric FMRP is similar to that in this study. However, the intermolecular disulfide bond, as well as the oligomerization state of FMRP in solution, was not observed and discussed. In this study, we successfully synthesized piMIPs, and infrared spectral analysis suggested the complete removal of the protein template, so there was no interference of the template in protein crystallization trials. To further test the advantages of piMIPs in promoting protein crystallization, five model proteins were used. From Table 1 , we found that protein crystals were observed in their cognate piMIPs and in some non-cognate piMIPs, MIP 0 and piNIPs, but were not observed in the NIP 0 and CK (without any polymers) under metastable conditions. This indicates excellent crystal-inducing characteristics of the cognate piMIPs, which are results of integrating MIPs and precipitants. By comparing the performance of piMIPs with MIP 0 and piNIPs with NIP 0 , we could validate that the immobilized precipitant was critical for enhancing crystal diffraction resolution, implying that piMIPs may help flexible regions tuning into ordered state and thus enhance the resolution. The success in obtaining high-quality FMRPΔ crystals provides direct evidence to support this point. By carefully comparing the performance of two series of piMIPs, we realized that certain relationships between immobilized precipitant and free precipitant was required. It is known that a protein needs a certain precipitant to promote crystallization [47] , and (NH 4 ) 2 SO 4 , NaCl and Na/K tartrate are small molecular inorganic salts. Thus, if the immobilized precipitant does not match or resemble the free precipitant, the energy barrier may not be reduced effectively. These results further attested the ability of the immobilized precipitant, whose efficacy was greatest when embedded with cognate piMIPs. In summary, we have incorporated conventional precipitants into MIPs to promote protein crystallization. We demonstrated piMIPs successful use in crystallization of flexible FMRPΔ and high-quality crystals were obtained regardless of solvent content (78%) and high flexibility. Surprisingly, a novel KH domain, KH0, and an intermolecular disulfide bond were identified for the first time. Our findings provide a structural basis for drug design in treating neurologic diseases and protecting against influenza. In addition, the precipitant best suited for solution conditions was also the optimal precipitant for use in the preparation of the cognate piMIPs. For five model proteins, piMIPs facilitated high-quality crystals formation when compared with other nucleants. For catalase, piMIPs can also grow crystals that were missed when using other nucleants. These piMIPs could perform key roles in assembling protein molecules to form high supersaturation states, stabilizing flexible loops and aid the growth of ordered crystals out of the solution, and inducing the formation of large single crystals. By immobilizing precipitants onto MIPs, we provide an effective way for optimal protein crystal growth, especially for many multi-domain proteins that can be extremely difficult to crystallize because of the inherent high flexibility of loops. Preparation of FMRP DNA fragments encoding various amino-acid segments of wild-type human FMRP (NCBI Reference Sequence: AGO02166) and mutants were amplified by PCR and ligated into a modified pET28a vector with a tobacco etch virus (TEV) protease cleavage site. The final clones were verified by restriction enzyme digestion and DNA sequencing. The proteins were overexpressed at 37 °C in Escherichia coli strain BL21 (DE3) grown to an OD 600 of ~0.8 in Luria-Bertani medium with 50 μg ml −1 of kanamycin. Protein expression was induced by the addition of isopropyl β- D -1-thiogalactopyranoside to a final concentration of 0.2 mM and cells were grown for a further 12 h at 16 °C. All of purification procedures were performed at 4 °C. Cells were harvested by centrifugation, resuspended in 20 mM Tris-HCl, pH 7.5, 500 mM NaCl, 20 mM imidazole and lysed by sonication. Debris was removed by centrifugation at 20,000 g for 1 h. The soluble supernatant fraction was incubated with a Ni 2+ -chelating column (GE Healthcare) for 45 min. His-tagged protein was eluted with elution buffer (20 mM Tris-HCl, pH 7.5, 500 mM NaCl, 300 mM imidazole). The N-terminal His-tag was removed by digestion with TEV protease. After TEV protease digestion, the sample was passed over a second Ni 2+ -chelating column (GE Healthcare) to remove the cleaved His-tag and TEV protease (which is also His-tagged). The FMRP sample was further purified by a Q Sepharose High performance column (GE Healthcare). Then the proteins were loaded onto a Superdex 200 column (GE Healthcare) with buffer (20 mM Tris-HCl, pH 7.5, 150 mM NaCl). Fractions containing the protein were pooled and concentrated to ~12 mg ml −1 for crystallization experiments. Preparation of precipitant-immobilized imprinted polymers AMPSN used for preparation of the piMIP 2 series was obtained by reacting 2-acrylamido-2-methyl-1-propanesulfonic acid (AMPS) with an ammonium hydroxide solution (mole ratio of 1:2) for 6 h at room temperature. AMPSN powder was attained following lyophilization of this reaction mixture. As shown in Supplementary Fig. 2 , for preparation of the piMIP 1 and piMIP 2 series, poly (ethylene glycol) methyl ether acrylate (0.5 mmol) containing a PEG group or AMPSN (0.5 mmol) bearing a sulfonic ammonium group on the side chain, 2-hydroxyethyl methacrylate (0.3 mmol) and N,N′-methylenebis (acrylamide) (MBA) (0.04 mmol) were dissolved in 300 μl of deionized water. Then 100 μl of the 12 mg ml −1 template protein solution was added and the mixture was incubated at 25 °C for 30 min. Subsequently, 20 μl of a 10% (w/v) ammonium persulphate solution was added and the solution was purged with nitrogen for 5 min. Then 20 μl 5% (v/v) N , N , N ′, N '-tetramethylethylenediamine solution was added and the solution was left to polymerize (18 h) at room temperature. Simultaneously, the corresponding piNIPs were also produced using the same procedure without the template. With the free radical polymerization, precipitants were immobilized onto the backbone of the obtained polymers. The polymers were then ground and washed using deionized water five times to remove unreacted monomer. To elute the template protein from the polymer, 10% AcOH:SDS solution was used to destroy the hydrogen bond interactions between the template protein and polymer. The template protein was removed completely and this removal was monitored until the infrared spectra of piMIPs and piNIPs were basically consistent. Finally, polymers were washed again with deionized water ten times to remove AcOH and SDS. The remaining piMIPs and piNIPs were stored at 4 °C. For the preparation of MIP 0 and NIP 0 , acrylamide (AM) (0.5 mmol), 2-hydroxyethyl methacrylate (0.3 mmol) and MBA (0.04 mmol) were used, and the detailed steps were similar to those used for piMIPs and piNIPs preparation. Particle size analysis of piMIPs and piNIPs L-piMIPs with the lowest molecule weight protein as template and C-piMIPs with the highest molecule weight protein as template were picked out for particle size analysis. The particle diameter and size distributions of L-piMIP 1 , L-piMIP 2 , C-piMIP 1 , C-piMIP 2 , piNIP 1 and piNIP 2 were measured using a laser-scattering particle size distribution analyser (LA-950, Horiba Ltd.). The experiments were carried out using deionized water to dilute the samples. The instrument settings were: refractive indexes of the deionized water and sample were 1.333 and 1.600, respectively. The data were obtained and analysed using the programme Horiba LA-950 for Windows (wet) ver 5.10. Particle size calculations were based on the Mie-Scattering theory. The mean, median, mode, diameter on cumulative and cumulative on diameter were obtained. And the median size and mean size were listed in Supplementary Table 1 . FT-IR spectrometry analysis of piMIPs and piNIPs FT-IR spectra were recorded on a spectrometer (TENSOR 27, Bruker, Germany) with KBr pellets at room temperature using an accumulation of 32 scans and a resolution of 4 cm −1 in the range of 4,000–400 cm −1 . Samples (2 mg) were thoroughly ground with KBr and pellets were prepared using a hydraulic press under a pressure of 600 kg cm −2 . Crystallization experiments For FMRPΔ, the hanging-drop vapour-diffusion method was used and 400 μl reservoir solution was added into the 24-well plate with 4 μl as the final drop volume (2.0 μl protein solution, 0.2 μl piMIPs, piNIPs, MIP 0 or NIP 0 and 1.8 μl reservoir solution). FMRPΔ and other constructs were dissolved in a solution containing 20 mM Tris-HCl (pH 7.5) and 150 mM NaCl with a final protein concentration of 12 mg ml −1 . For the preliminary screen, crystallization was performed at 18 and 4 °C by the sitting-drop vapour-diffusion method using Crystal Screen, Crystal Screen 2, Crystal Screen HT, Index, Index HT crystallization kits from Hampton Research. Fortunately, initial crystals were found after about 20 days at 18 °C with a buffer containing 100 mM BIS-TRIS propane (BTP) (pH 7.0) and 2 M HCO 2 Na. However, the numerous crystals in one droplet were miniscule. Consequently, gradients of precipitant concentration and pH were screened in 18 and 4 °C, and 23 different salts and 7 different buffers were also screened. Larger crystals were obtained in conditions which contained 100 mM Bis-Tris, pH 7.0, 1.8 M HCO 2 Na at 18 °C, but they were fragile and clustered. X-ray diffraction tests gave low-resolution (~10 Å). In consideration of the high tendency to aggregate and high flexibility of FMRPΔ, an additive screen and a detergent screen (Hampton research) were carried out; however, the results did not lead to better quality crystals. piMIPs were then used to crystallize FMRPΔ. Crystals were screened by the hanging-drop method by mixing 1.8 μl reservoir buffer plus 0.2 μl piMIPs with 2 μl protein solution under the same conditions: 100 mM Bis-Tris, pH 7.0, 1.8 M HCO 2 Na at 18 °C. Finally, high-quality crystals were obtained after 2 weeks at 18 °C in the presence of F-piMIP 2 . The X-ray diffraction resolution increased to 3 Å. All the crystals were transferred to a cryo-buffer (reservoir buffer supplemented with 25% ethylene glycol) and were immediately frozen in liquid nitrogen before data collection. For the five model proteins, the sitting-drop vapor-diffusion method was used for the crystallization of lysozyme, catalase, trypsin, proteinase K and glucose isomerase. One microlitre protein solution was mixed with 1 μl reservoir solution, and then 0.2 μl aliquot of piMIPs, piNIPs, MIP 0 or NIP 0 was dispensed with a pipet into the drops. Conditions tested for the proteins were as follows: lysozyme at 20 mg ml −1 : from 2% (w/v) to 3% (w/v) NaCl, all in 0.1 M NaAc buffer with pH 4.5. The metastable conditions referred in Table 1 corresponding to 2.5% (w/v) NaCl. Trypsin was dissolved in the solution of 10 mg ml −1 of benzamidine and 3 mM CaCl 2 to give a final protein solution of 30 mg ml −1 . The composition of reservoir solution was set from 1.0 to 2.4 M (NH 4 ) 2 SO 4 , all buffered in 0.1 M Tris-HCl at pH 8.5. The metastable conditions referred in Table 1 corresponding to 1.6 M (NH 4 ) 2 SO 4 . Proteinase K (20 mg) was dissolved in 1 ml of solution of 1 mM phenylmethylsulphonyl fluoride and 25 mM HEPES (pH 7.0). Crystallization conditions were from 0.025 to 0.6 M Na/K tartrate, all in 1 mM phenylmethylsulphonyl fluoride and 25 mM HEPES at pH 7.0. And the metastable condition referred in the Table 1 was at 0.05 M Na/K tartrate. Glucose isomerase at 33 mg ml −1 : from 0.25 to 2.5 M (NH 4 ) 2 SO 4 pH 7.0. And the metastable condition in the Table 1 was referred to 0.5 M (NH 4 ) 2 SO 4 . Catalase at 12 mg ml −1 : from 5 to 10% (w/v) PEG 6 K, 5% (v/v) 2-methyl-2,4-pentadiol (MPD) in 0.1 M Tris-HCl buffer (pH 7.5). The metastable condition referred in Table 1 was corresponding to 6% (w/v) PEG 6 K. Diffraction data collection and structure determination For model proteins, data were collected on beamline BL17U1 at the Shanghai Synchrotron Radiation Facility or NE3A at the Photon Factory (KEK). For FMRPΔ, native data were collected on beamline NE3A at the Photon Factory. Data were indexed, integrated and scaled with the HKL2000 suite of programmes [48] . Initial attempts to solve the FMRPΔ structure by any molecular replacement programmes using the FMRP (residues: 1−134, PDB accession number 2BKD ) NMR structure [5] as the search model failed. This may be because of the high flexibility of the FMRP structure. After extensive trials of different models, an initial solution was obtained by the molecular replacement programme BALBES [49] using the structure of FXR1 (PDB accession number 3O8V ) [21] as the model, with an MR score of 10.27 and R work / R free values 38.3%/42.1% with the space group C2. The inappropriate main and side chains were removed in the density map by the programme COOT [50] and REFAMC5 (ref. 51 ) was used to refine the model. After numerous cross revisions, the best model was only refined to give R work / R free values of 33.5%/37.2%. Based on these results, we tried using the programme package of IPCAS [52] within the CCP4 suite [53] . The final structure was refined to 3.0 Å with an R work of 21.9% and an R free of 25.9%. The crystal contains four protein molecules per asymmetric unit, giving a crystal solvent content of 78%. Data collection and processing statistics are shown in Table 2 . All structural figures were made using PyMOL. Analytical ultracentrifugation SV experiments were performed in a Beckman/Coulter XL-I analytical ultracentrifuge using double-sector or six-channel centerpieces and sapphirine windows. An additional protein purification step involving the use of size exclusion chromatography in a buffer containing 20 mM Tris-HCl, pH 7.5, 150 mM NaCl was performed before the experiments. SV experiments were conducted at 42,000 r.p.m. and 4 °C using interference detection and double-sector cells loaded at approximate 0.2 mM for FMRPΔ and the C99S Mutant. The buffer composition (density and viscosity) and protein partial specific volume (V-bar) were obtained using the programme SEDNTERP. The SV data were analysed using the SEDFIT programmes [54] . Size exclusion chromatography The FMRPΔ WT or mutants were applied to a Superdex-75 10/300 column (GE Healthcare) equilibrated with a buffer containing 20 mM Tris-HCl, pH 7.5 and 150 mM NaCl. To compare the different elution volumes between FMRPΔ wild-type, C99S, I106A and the M183A/L184A/D186A/M187A quadruple mutant, ~7 mg of protein was loaded onto the Superdex-75 column. The proteins were visualized by SDS–polyacrylamide gel electrophoresis followed by Coomassie blue staining. SAXS experiments SAXS data were collected at the BioSAXS station (1W2A) of the BSRF, using previously published methods [55] . Briefly, the FMRPΔ wild-type and the C99S mutant were subjected to size exclusion chromatography with a buffer containing 20 mM Tris-HCl, pH 7.5, and 150 mM NaCl. The protein concentrations were 5 mg ml −1 (about 0.22 mM), and the data of the protein samples were collected at 1.54 Å with a distance of 1.64 m from the detector. Data collection time of 5 min was used for all samples split into two 150 s time frames to assess and remove effects from radiation damage to the samples. Individual data were processed by FIT2D [56] . The scattering from the buffer alone was measured before and after each sample measurement and the average of the scattering before and after each sample was used for background subtraction. The theoretical scattering curves from three possible configurations of FMRPΔ or its mutant were fitted to the experimental scattering curve using the MES algorithm [28] . Accession codes: Final coordinates of the human FMRPΔ structure has been deposited in the Protein Data Bank (PDB ID code 4OVA ). How to cite this article: Hu, Y. et al . The amino-terminal structure of human fragile X mental retardation protein obtained using precipitant-immobilized imprinted polymers. Nat. Commun. 6:6634 doi: 10.1038/ncomms7634 (2015).